ArabidopsisSABREandCLASPinteract to stabilize cell division plane orientation and planar polarity The orientation of cell division and the coordination of cell polarity within the plane of the tissue layer (planar polarity) contribute to shape diverse multicellular organisms. The root of Arabidopsis thaliana displays regularly oriented cell divisions, cell elongation and planar polarity providing a plant model system to study these processes. Here we report that the SABRE protein, which shares similarity with proteins of unknown function throughout eukaryotes, has important roles in orienting cell division and planar polarity. SABRE localizes at the plasma membrane, endomembranes, mitotic spindle and cell plate. SABRE stabilizes the orientation of CLASP-labelled preprophase band microtubules predicting the cell division plane, and of cortical microtubules driving cell elongation. During planar polarity establishment, sabre is epistatic to clasp at directing polar membrane domains of Rho-of-plant GTPases. Our findings mechanistically link SABRE to CLASP-dependent microtubule organization, shedding new light on the function of SABRE-related proteins in eukaryotes. Diverse multicellular organisms coordinate the polarity of single cells within the plane of the tissue layer [1] , [2] , [3] , [4] , [5] . This type of tissue polarity is commonly referred to as planar polarity [1] , [2] , [4] . The establishment of planar polarity is intensively studied for animal epithelia where Drosophila wing-hair polarization provides an invaluable model system [1] , [2] . Similarly, plants like Arabidopsis display planar polarity of coordinated polar hair outgrowth from root epidermal cells [3] , [4] and orientation of leaf epidermal hairs (trichomes) [5] . The upstream molecular mechanisms that direct planar polarity, however, differ substantially between animals and plants. In Drosophila , Wingless and its homologue dWnt4 act as long-range polarizing cues upstream of the Frizzled planar cell polarity pathway [6] , which transmits directional information to downstream effectors such as small Rho/Rac-type family GTPases [1] , [2] . By contrast, plants lack genes with similarity to Wnts or to core components of the Frizzled planar cell polarity pathway. Instead, planar polarity of root epidermal cells is coordinated by a tissue concentration gradient of the plant hormone auxin [4] , [7] . This gradient instructs the coordinated polar placement of hairs and of Rho-of-plant (ROP) GTPases that mark the initiation of planar polarity of root hair positioning before morphological hair outgrowth [4] , [7] . ROP2/4 localization provides the earliest read-out for polar hair initiation [8] , [9] and regulation of ROP activity spatially restricts polar root hair initiation [9] , [10] . During morphogenesis of leaf pavement cells, auxin can activate ROP2/4 and ROP6 to differentially organize the actin and tubulin cytoskeleton, respectively [11] , [12] . Actin and tubulin are also required for planar polarity of root hair initiation [13] , [14] , but cytoskeletal dynamics and their regulation remain uncharacterized during this process. Similarly, the sole microtubule-associated protein known to be required for planar orientation of leaf trichomes is the CLIP170-associated protein (CLASP) from Arabidopsis [15] . Further, CLASP mediates orientation of cell division planes in roots [16] , [17] , modulates the abundance [18] , [19] as well as the polarity of PIN2 protein in root cortical cells [19] , and CLASP homologues regulate cellular asymmetries in other eukaryotes [20] . At the molecular level, CLASP homologues associate with and stabilize the plus ends of dynamic microtubules [20] , stabilize microtubule arrays during cell division [15] , [16] , [20] and promote microtubule growth around cell edges contributing to the generation of plant cortical microtubule arrays [21] . Here we report new functions for the Arabidopsis SABRE ( SAB ) gene, mechanistically linking its action to CLASP-mediated microtubule organization. We thus unravel new interactions contributing to the framework of cell division plane orientation and planar polarity formation in plants. Our findings may help to elucidate the function of uncharacterized SAB-like proteins found throughout eukaryotes and their potential function in cytoskeletal organization during cell division, cell morphogenesis and its coordination. kreuz und quer affects cell and planar polarity The root hairs of Arabidopsis regularly emerge from the outer membrane of epidermal cells and coordinately initiate close to, albeit not completely at, the root tip-oriented (basal) ends of cells ( Fig. 1a ). As knowledge about genes contributing to planar polarity in plants remains limited, we performed a genetic screen for root hair-positioning mutants to identify additional factors. This led to the identification of the recessive kreuz und quer ( kuq ) mutant generated by fast neutron mutagenesis. kuq displayed a more random distribution of hair position towards both the basal and the apical ends of cells ( Fig. 1b,c ). We also observed the localization of polar ROP protein patches at the outer membrane of root hair cells before morphological hair outgrowth. Unlike wild type ( Fig. 1d ), kuq mutant cells often showed more basal or apical localization of ROP ( Fig. 1e–g ). In contrast, the polar distribution of PEN3-GFP ( Supplementary Fig. S1a,b ) that broadly defines the outer membrane [22] , [23] as well as the apical polarity of the PIN2 auxin efflux carrier ( Supplementary Fig. S1c,d ) remained largely unaffected in root epidermal cells of kuq ( Supplementary Fig. S1b,d ). More strikingly, the polarity of GFP-BASL [24] , which almost invariably localizes to basal membranes and to nuclei when ectopically expressed in wild-type root epidermal cells (99.8% basal, 0.2% of cells apical localization; n =514) was significantly more often switched to apical ends of epidermal cells in kuq (8.6% of cells with apical localization; n =187; P =5.1 × 10 −9 by Fisher’s exact test; Supplementary Fig. S1e, f ). These findings suggest that kuq affects basal membrane polarity and basal bias of planar polarity rather than outer lateral membrane polarity in the root epidermis. 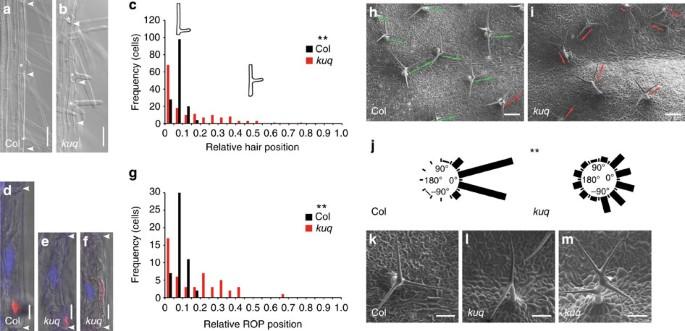Figure 1:kuqmutation affects epidermal cell and planar polarity. (a,b) Hair-forming root epidermal cells of 5-day-old (a) wild-type Columbia (Col) and (b)kuqseedlings. Arrowheads, apical and basal ends of cells ina,bandd–f. Asterisks indicate sites of hair formation inaandb. (c) Quantitative analysis of planar polarity phenotypes as relative root hair position in Col andkuq. Number of cells in classes (frequency) with hair positions are indicated between basal (0) and apical (1) ends of cells (**P=0.000 Col versuskuq, determined by non-parametric, two-sample Kolmogorov–Smirnov (K–S) test,n=150 cells from 30 roots per genotype). (d–f) anti-ROP (red) immunofluorescence in Col, (e,f)kuqepidermal cells, combined with DAPI-stained nuclei (blue) and brightfield microscopy image. (g) Quantitative analysis of planar polarity phenotypes of ROP protein patch positions along apical-basal axis of epidermal cells in Col andkuq. Number of cells in classes (frequency) showing ROP positions between basal (0) and apical (1) ends is shown (**P=0.000 Col versuskuqby K–S test,n=50 cells per genotype, from 10 Col and 19kuqroots). (h,i,k–m) Scanning electron microscopy (SEM) images of leaf trichomes of (h,k) Col, (i,l,m)kuq-mutant leaves. (h,i) Planar polarity of first trichome branch orientation along proximo-distal leaf axis (arrows). Distal ends of leaves are to the left, proximal ends to the right. Deviation of <30° and >30° from proximal orientation is indicated by green and red arrows, respectively. (j) Quantitative analysis of first trichome branch orientation from SEM images of Col andkuq. 0° indicates proximal orientation, 180° distal orientation of trichome branches. (**P<0.001 Col versuskuqby F-test,n=174 trichomes per genotype). (k–m) Trichome branching phenotypes of (k) Col and (l,m)kuq. Note, (l) trichomes with two branches or (m) additional ectopically placed branch inkuq(arrowhead). For statistical analysis, seeFig. 5a. Scale bars, 50 μm (a,b), 10 μm (d–f), 200 μm (h,i), 100 μm (k–m). Figure 1: kuq mutation affects epidermal cell and planar polarity. ( a , b ) Hair-forming root epidermal cells of 5-day-old ( a ) wild-type Columbia (Col) and ( b ) kuq seedlings. Arrowheads, apical and basal ends of cells in a , b and d – f . Asterisks indicate sites of hair formation in a and b . ( c ) Quantitative analysis of planar polarity phenotypes as relative root hair position in Col and kuq . Number of cells in classes (frequency) with hair positions are indicated between basal (0) and apical (1) ends of cells (** P =0.000 Col versus kuq , determined by non-parametric, two-sample Kolmogorov–Smirnov (K–S) test, n =150 cells from 30 roots per genotype). ( d – f ) anti-ROP (red) immunofluorescence in Col, ( e , f ) kuq epidermal cells, combined with DAPI-stained nuclei (blue) and brightfield microscopy image. ( g ) Quantitative analysis of planar polarity phenotypes of ROP protein patch positions along apical-basal axis of epidermal cells in Col and kuq . Number of cells in classes (frequency) showing ROP positions between basal (0) and apical (1) ends is shown (** P =0.000 Col versus kuq by K–S test, n =50 cells per genotype, from 10 Col and 19 kuq roots). ( h , i , k – m ) Scanning electron microscopy (SEM) images of leaf trichomes of ( h , k ) Col, ( i , l , m ) kuq -mutant leaves. ( h , i ) Planar polarity of first trichome branch orientation along proximo-distal leaf axis (arrows). Distal ends of leaves are to the left, proximal ends to the right. Deviation of <30° and >30° from proximal orientation is indicated by green and red arrows, respectively. ( j ) Quantitative analysis of first trichome branch orientation from SEM images of Col and kuq . 0° indicates proximal orientation, 180° distal orientation of trichome branches. (** P <0.001 Col versus kuq by F-test, n =174 trichomes per genotype). ( k – m ) Trichome branching phenotypes of ( k ) Col and ( l , m ) kuq . Note, ( l ) trichomes with two branches or ( m ) additional ectopically placed branch in kuq (arrowhead). For statistical analysis, see Fig. 5a . Scale bars, 50 μm ( a , b ), 10 μm ( d – f ), 200 μm ( h , i ), 100 μm ( k – m ). Full size image Leaf trichome orientation provides another model for the analysis of both cell and planar polarity. Arabidopsis wild-type trichomes predominantly carry three branches, and the first branch, initiating closest to the leaf surface, is oriented towards the proximal end of the leaf [5] , [15] providing a planar polarity read-out. Intriguingly, orientation of the first branch proved much more variable in the kuq mutant than in the wild type ( Fig. 1h–j ), revealing defective planar polarity of trichome orientation. At the cellular level, kuq mutant leaves showed two-branched trichomes more often than wild-type leaves ( Fig. 1k,l ; for quantitative analysis see below) and sometimes displayed irregular placement of branches along the trichome stalk ( Fig. 1m ). The reduction in branch number and the ectopic placement of branches on trichomes in kuq indicated a cell polarity defect in the initiation and placement of trichome branches. Interestingly, reduced trichome branch number has been reported for Arabidopsis mutants defective in tubulin and microtubule-associated proteins [25] . Hence, kuq affects cell and planar polarity in leaf and root epidermis, causing phenotypes characteristic of microtubule cytoskeleton mutants. kuq is allelic to SABRE We mapped the kuq mutation to a 480-kb interval on chromosome 1 by positional cloning ( Fig. 2 ) and analysed phenotypes of T-DNA insertion lines in candidate genes within this interval. Homozygous seedlings from 9 out of 11 T-DNA insertion lines in one of these genes, SABRE ( SAB ) (At1g58250; Fig. 2 ) displayed phenotypes indistinguishable from that of kuq , whereas two showed similar but weaker seedling root and adult shoot defects ( Figs 2 and 3a ). Sequencing of the genomic SAB coding region in kuq identified a single-nucleotide deletion at position 6,592 (of 7,824), predicted to induce a nonsense mutation generating a premature stop codon ( Fig. 2 ). Other SAB -mutant alleles have been described to display anisotropic expansion of root cortical cells [26] , [27] , [28] or an enhanced response to phosphate starvation [29] . More detailed analysis of three SAB T-DNA insertion lines, SALK 108709 ( sab-5 ), SALK 52995 ( sab-6 ) and SALK 123771 ( sab-7 ) uncovered reduced epidermal cell length and defective planar polarity of root-hair position similar to that of the kuq mutant ( Fig. 3b–e ). Complementation analyses revealed that these three lines were allelic to kuq and to each other and they are, therefore, in the following referred to as sab kuq , sab-5 , sab-6 and sab-7. The sab-7 mutant carrying an insertion into the second last exon of the SAB gene ( Fig. 2 ) was somewhat less affected, identifying it as a hypomorphic allele ( Fig. 3a,b,e ). Reverse transcription PCR (RT–PCR) analyses revealed that neither sab-5 , sab-6 nor sab-8 (SALK 12897) produced a full-length transcript, in contrast to sab kuq for which a transcript could be detected when using primers spanning the region including the single-nucleotide deletion ( Fig. 3f–h ). We subsequently employed sab-5 in parallel to or instead of sab kuq because sab-5 carried the T-DNA insertion closest to the 5′-end of the SAB coding region ( Fig. 2 ), did not express full-length SAB complementary DNA (cDNA) ( Fig. 3f–h ) and displayed phenotypic defects similar to sab kuq ( Fig. 3a–c , Supplementary Fig. S2a–l ). Thus, cloning of sab kuq revealed a central role for SAB in cell and planar polarity. 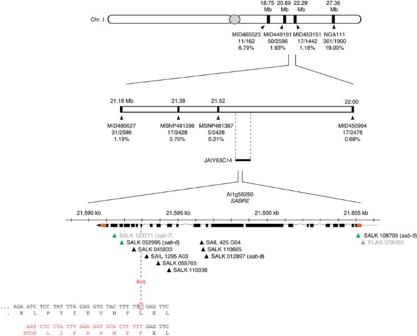Figure 2:kuqcauses a single-nucleotide deletion in theSABREgene. Map-based identification of thekuqmutation in theSABgene. Simple-sequence-length polymorphism (SSLP; NGA111), custom-made SSLPs (Monsanto Insertion/Deletion polymorphism; MID) and custom-made cleaved amplified polymorphic sequence (CAPS; MSNP) markers are indicated with respective position, recombinant/total chromosomes and recombination frequency. Digits of MID and MSNP markers correspond to polymorphism accession number in MonsantoArabidopsisPolymorphism Collection (http://www.arabidopsis.org/browse/Cereon/index.jsp). Note the 480-kb mapping interval containing JAtY63C14 transformation-competent bacterial artificial chromosome carrying theSABgene. Insertion positions of 11SABT-DNA lines analysed are indicated by arrowheads below the gene structure. Black boxes, exons; lines, introns; orange boxes, untranslated regions. T-DNA lines in black, homozygous seedlings phenotypically indistinguishable fromkuqmutants; T-DNA lines in grey, weaker phenotype. T-DNA lines with green arrowheads, tested for allelism tokuqby complementation test. Red circle, cytosine deletion inkuqinducing a premature stop codon in 17th exon ofSAB; upper rows, wild-type coding sequence and amino-acid translation; lower rows,kuq. Figure 2: kuq causes a single-nucleotide deletion in the SABRE gene. Map-based identification of the kuq mutation in the SAB gene. Simple-sequence-length polymorphism (SSLP; NGA111), custom-made SSLPs (Monsanto Insertion/Deletion polymorphism; MID) and custom-made cleaved amplified polymorphic sequence (CAPS; MSNP) markers are indicated with respective position, recombinant/total chromosomes and recombination frequency. Digits of MID and MSNP markers correspond to polymorphism accession number in Monsanto Arabidopsis Polymorphism Collection ( http://www.arabidopsis.org/browse/Cereon/index.jsp ). Note the 480-kb mapping interval containing JAtY63C14 transformation-competent bacterial artificial chromosome carrying the SAB gene. Insertion positions of 11 SAB T-DNA lines analysed are indicated by arrowheads below the gene structure. Black boxes, exons; lines, introns; orange boxes, untranslated regions. T-DNA lines in black, homozygous seedlings phenotypically indistinguishable from kuq mutants; T-DNA lines in grey, weaker phenotype. T-DNA lines with green arrowheads, tested for allelism to kuq by complementation test. Red circle, cytosine deletion in kuq inducing a premature stop codon in 17th exon of SAB ; upper rows, wild-type coding sequence and amino-acid translation; lower rows, kuq . 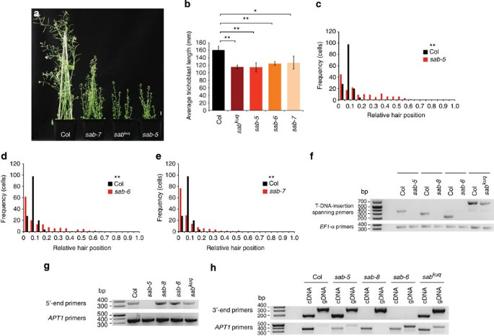Figure 3: Phenotypic and RT–PCR analyses of additionalSABT-DNA-mutant alleles. (a) Five-week-old plants of Col,sab-7,sabkuqandsab-5. Note,sab-5is indistinguishable fromsabkuqwhilesab-7is less affected. (b) Quantitative analysis of trichoblast length in Col andSAB-mutant alleles. Average cell length ofn=150 trichoblasts from 30 roots per genotype. Data are means±s.d. fromn=3 independent experiments. Statistical differences determined by two-tailed, unpairedt-test with equal variance and significance levelP<0.05 are indicated as *P<0.05 and **P<0.01;n=3. Allsaballeles differ significantly from wild type but do not differ from each other (P>0.05). (c–e) Quantitative analysis of planar polarity defects in (c)sab-5, (d)sab-6and (e)sab-7compared with Col is displayed as relative root hair position similar toFig. 1c. **P=0.000 Col versussab-5,sab-6orsab-7by K–S test,n=150 cells from 30 roots per genotype. (f–h) Semiquantitative RT–PCR analysis of wild-type Col andsab-mutant seedlings.SABtranscript was amplified with (f) primers spanning the T-DNA insertion (or single-nucleotide deletion) and primers located close to (g) the 5′- or (h) the 3′-end ofSABcoding sequence. Primers close to 3′-end were also employed on genomic DNA (gDNA) extracted from the same plant material used for cDNA (cDNA) synthesis. PartialSABtranscripts were detected in all T-DNA alleles.EF1-αandAPT1were utilized as controls. Scale bar, 10 mm. Full size image Figure 3: Phenotypic and RT–PCR analyses of additional SAB T-DNA-mutant alleles. ( a ) Five-week-old plants of Col, sab-7 , sab kuq and sab-5 . Note, sab-5 is indistinguishable from sab kuq while sab-7 is less affected. ( b ) Quantitative analysis of trichoblast length in Col and SAB -mutant alleles. Average cell length of n =150 trichoblasts from 30 roots per genotype. Data are means±s.d. from n =3 independent experiments. Statistical differences determined by two-tailed, unpaired t -test with equal variance and significance level P <0.05 are indicated as * P <0.05 and ** P <0.01; n =3. All sab alleles differ significantly from wild type but do not differ from each other ( P >0.05). ( c – e ) Quantitative analysis of planar polarity defects in ( c ) sab-5 , ( d ) sab-6 and ( e ) sab-7 compared with Col is displayed as relative root hair position similar to Fig. 1c . ** P =0.000 Col versus sab-5 , sab-6 or sab-7 by K–S test, n =150 cells from 30 roots per genotype. ( f – h ) Semiquantitative RT–PCR analysis of wild-type Col and sab -mutant seedlings. SAB transcript was amplified with ( f ) primers spanning the T-DNA insertion (or single-nucleotide deletion) and primers located close to ( g ) the 5′- or ( h ) the 3′-end of SAB coding sequence. Primers close to 3′-end were also employed on genomic DNA (gDNA) extracted from the same plant material used for cDNA (cDNA) synthesis. Partial SAB transcripts were detected in all T-DNA alleles. EF1-α and APT1 were utilized as controls. Scale bar, 10 mm. Full size image SABRE-like proteins in other eukaryotes Our sequencing of SAB wild-type cDNA amplified from Arabidopsis roots experimentally verified the presence of an 8,347-bp transcript encoding a 2,607 amino acid protein identical to the predicted protein sequence At1g58250.1 (ref. 29 ). Depending on the transmembrane helix prediction algorithm employed, SAB is predicted to contain one (TMHMM, Pred-TMR), two (TMpred) or three transmembrane domains (TopPred2, HMMTOP). All programs predict the first six to eight amino-terminal amino acids preceding the first transmembrane domain to be cytosolic. This indicates that SAB contains an internal, hydrophobic start-transfer sequence rather than an N-terminal cleavable signal peptide and that SAB may be a transmembrane protein rather than a secreted protein. Proteins with sequences related to the predicted 2,607 amino acid SAB protein are found throughout diverse eukaryotes ( Fig. 4a ). In Arabidopsis thaliana , KINKY POLLEN (KIP) shares the highest sequence identity with SABRE [28] . Although plant species harbour either one or two SAB -like genes in their genomes, all animal genomes analysed, including the human and mouse genomes, possess a single-copy gene encoding a protein of similar size with highest sequence identity restricted to two larger protein regions ( Fig. 4b ). To date, none of the genes related to SAB from non-plant eukaryotes has been functionally characterized. However, mutants defective in the Arabidopsis KIP gene and the closely related ABERRANT POLLEN TRANSMISSION1 (APT1) gene from maize are defective in pollen tube growth [28] , [30] . APT1 , like SAB , codes for a predicted 2,607 amino acid protein [30] . When transiently expressed in tobacco pollen, a carboxy-terminal 108 amino acid peptide from APT1 fused to green fluorescent protein (GFP) localizes to the Golgi apparatus [30] . The peptide has been annotated as a Golgi-body localization domain in the conserved domain database [31] . However, although SAB is a predicted membrane protein with the N terminus oriented towards the cytosol, the biological and molecular function of SAB and related proteins as well as the subcellular localization of full-length proteins remain to be addressed in any eukaryote. 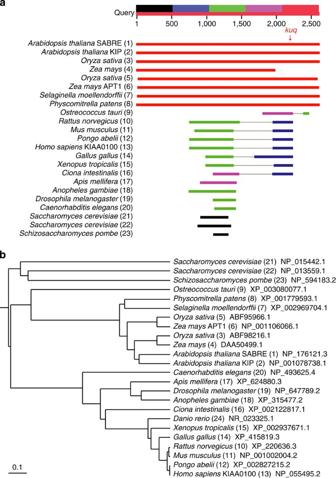Figure 4: SAB-related proteins in diverse eukaryotes. (a) Blastp search for proteins homologous to SAB and alignment of SAB-like protein sequences from selected organisms. Note, sequence similarity with proteins from more distantly related species is restricted to two distinct regions of about 600 and 300 amino acids. Red arrow, position of premature stop codon introduced bykuqmutation. Numbers in parentheses refer to sequences inb. Red, alignments with highest sequence identity; black, lowest sequence identity. (b) Phylogenetic tree based on sequences of SAB-related proteins in selected species, showing evolutionary conservation of SAB across a wide variety of eukaryotic organisms. NCBI reference sequence or GenBank accession number for each protein are indicated next to the respective species. Figure 4: SAB-related proteins in diverse eukaryotes. ( a ) Blastp search for proteins homologous to SAB and alignment of SAB-like protein sequences from selected organisms. Note, sequence similarity with proteins from more distantly related species is restricted to two distinct regions of about 600 and 300 amino acids. Red arrow, position of premature stop codon introduced by kuq mutation. Numbers in parentheses refer to sequences in b . Red, alignments with highest sequence identity; black, lowest sequence identity. ( b ) Phylogenetic tree based on sequences of SAB-related proteins in selected species, showing evolutionary conservation of SAB across a wide variety of eukaryotic organisms. NCBI reference sequence or GenBank accession number for each protein are indicated next to the respective species. Full size image SAB – CLASP interaction in planar polarity As the SAB sequence did not provide information about the molecular function of the protein, we addressed the mechanism of SAB action by analysing its genetic interactions. The combination of trichome branching and orientation defects observed in sab mutants had been described for clasp mutants [15] . We therefore generated a sab-5;clasp-1 double mutant and observed a strongly enhanced trichome branching defect, when compared with the respective single mutants or sab kuq ( Fig. 5a ; Supplementary Fig. S3a,b ), suggesting that SAB and CLASP synergistically interact during placement of trichome branches. Similarly, root length and overall growth of sab-5;clasp-1 double-mutant seedlings was severely reduced compared with the single mutants, further pointing towards a synergistic interaction at this level ( Fig. 5b ; Supplementary Fig. S3c ). 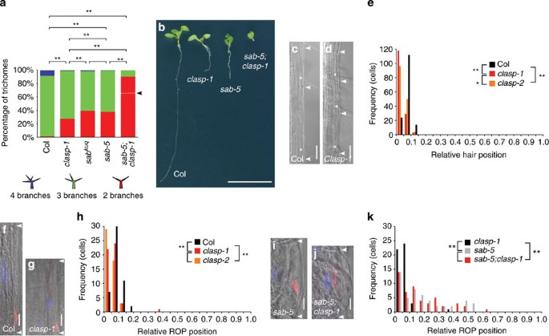Figure 5:SAB–CLASPinteraction mediates planar polarity upstream of ROP. (a–k) Genetic action ofsaband interaction withclaspduring (a) leaf trichome branching, (b) seedling development and (c–k) planar root epidermal polarity establishment. (a) Percentage of 2-branched (red), 3-branched (green) and 4-branched (blue) trichomes in Col (total trichome number:n=545),clasp-1(n=537),kuq-mutant allele ofSAB(sabkuq;n=409),sab-5(n=498) andsab-5;clasp-1(n=431) obtained from 10–16 leaves per genotype. Note, significant differences between all genotypes except forsab-5andsabkuq(P=0.51); the percentage of 2-branched trichomes insab-5;clasp-1highly significantly differed from the sum of the respective single-mutant values (dotted line, arrowhead;P<0.001). Significances were determined by Fisher’s exact test with significance levelP<0.05 and are indicated as **P<0.01.Supplementary Table S1shows exactP-values. (b) Ten-day-old Col,clasp-1,sab-5andsab-5;clasp-1seedlings. (c,d) Root hair position on epidermal cells of 5-day-old (c) Col and (d)clasp-1seedlings. (e) Quantitative analysis of planar polarity in Col,clasp-1andclasp-2is displayed as relative root hair position as inFig. 1c. (**P=0.000 Col versusclasp-1; **P=0.000 Col versusclasp-2by K–S test;n=150 cells per genotype). (f,g,i,j) Planar polarity phenotypes revealed by anti-ROP immunolabelling (red), DAPI (blue) overlaid with brightfield image of epidermal cells from (f) Col, (g)clasp-1, (i)sab-5and (j)sab-5;clasp-1. (h,k) Quantitative analysis of polar ROP protein patch positions as inFig. 1g. (h) Col,clasp-1,clasp-2, (k)clasp-1, sab-5andsab-5;clasp-1(**P=0.004 Col versusclasp-1; **P=0.000 Col versusclasp-2;P=0.241clasp-1versusclasp-2; **P=0.000clasp-1versussab-5; **P=0.000clasp-1versussab-5;clasp-1;P=0.841sab-5versussab-5;clasp-1by K–S test,n=50 cells from 8 to 22 roots per genotype). Arrowheads, apical and basal ends of cells inc,d,f,g,iandj. Asterisks indicate sites of hair formation incandd. Scale bars, 10 mm (b), 50 μm (c,d), 10 μm (f,g,i,j). Figure 5: SAB–CLASP interaction mediates planar polarity upstream of ROP. ( a – k ) Genetic action of sab and interaction with clasp during ( a ) leaf trichome branching, ( b ) seedling development and ( c – k ) planar root epidermal polarity establishment. ( a ) Percentage of 2-branched (red), 3-branched (green) and 4-branched (blue) trichomes in Col (total trichome number: n =545), clasp-1 ( n =537), kuq -mutant allele of SAB ( sab kuq ; n =409), sab-5 ( n =498) and sab-5;clasp-1 ( n =431) obtained from 10–16 leaves per genotype. Note, significant differences between all genotypes except for sab-5 and sab kuq ( P =0.51); the percentage of 2-branched trichomes in sab-5;clasp-1 highly significantly differed from the sum of the respective single-mutant values (dotted line, arrowhead; P <0.001). Significances were determined by Fisher’s exact test with significance level P <0.05 and are indicated as ** P <0.01. Supplementary Table S1 shows exact P -values. ( b ) Ten-day-old Col, clasp-1 , sab-5 and sab-5;clasp-1 seedlings. ( c , d ) Root hair position on epidermal cells of 5-day-old ( c ) Col and ( d ) clasp-1 seedlings. ( e ) Quantitative analysis of planar polarity in Col, clasp-1 and clasp-2 is displayed as relative root hair position as in Fig. 1c . (** P =0.000 Col versus clasp-1 ; ** P =0.000 Col versus clasp-2 by K–S test; n =150 cells per genotype). ( f , g , i,j ) Planar polarity phenotypes revealed by anti-ROP immunolabelling (red), DAPI (blue) overlaid with brightfield image of epidermal cells from ( f ) Col, ( g ) clasp-1 , ( i ) sab-5 and ( j ) sab-5;clasp-1 . ( h , k ) Quantitative analysis of polar ROP protein patch positions as in Fig. 1g . ( h ) Col, clasp-1 , clasp-2 , ( k ) clasp-1, sab-5 and sab-5;clasp-1 (** P =0.004 Col versus clasp-1 ; ** P =0.000 Col versus clasp-2 ; P =0.241 clasp-1 versus clasp-2 ; ** P =0.000 clasp-1 versus sab-5 ; ** P =0.000 clasp-1 versus sab-5;clasp-1 ; P =0.841 sab-5 versus sab-5;clasp-1 by K–S test, n =50 cells from 8 to 22 roots per genotype). Arrowheads, apical and basal ends of cells in c , d , f , g , i and j . Asterisks indicate sites of hair formation in c and d . Scale bars, 10 mm ( b ), 50 μm ( c , d ), 10 μm ( f , g , i , j ). Full size image We next addressed whether CLASP acts on planar polarity of root hair placement and observed a clear basal shift of hair position in clasp -mutant alleles ( Fig. 5c–e ). Similarly, ROP protein patches were misplaced towards the basal-most ends of elongating clasp -mutant epidermal cells when compared with the wild type ( Fig. 5f–h ), demonstrating that CLASP acts on planar polarity before ROP positioning. Strikingly, ROP positioning in sab-5;clasp-1 double-mutant seedlings was indistinguishable from that of sab-5 ( Fig. 5i–k ), suggesting that sab is epistatic to clasp during polar ROP positioning. SAB – CLASP interaction during division plane orientation The genetic interactions between SAB and CLASP prompted us to investigate whether SAB contributes to other processes that involve CLASP function, such as orientation of the cell division plane. Strikingly, sab-5- and sab kuq -mutant root meristems displayed strongly aberrantly orientated cell division planes when compared with the wild type ( Fig. 6a,b ; Supplementary Fig. S3d,e ). Live imaging of microtubules and nuclear DNA co-visualized by mCherry-TUBULIN ALPHA-5 (mCherry-TUA5) [32] , [33] and HISTONE2B-YELLOW FLUORESCENT PROTEIN (H2B-YFP) [34] , respectively, revealed that in comparison with wild type ( Fig. 6c ), sab-5 -mutant cells displayed misorientation of the preprophase band (PPB; Fig. 6d ). This orientation defect was followed by similarly misaligned spindle and phragmoplast orientation throughout mitosis and cytokinesis, whereas the overall timing of mitosis and cytokinesis was indistinguishable from wild-type root cells ( Fig. 6d ; Supplementary Movies 1 and 2 ). Similar results were obtained in immunolocalization studies demonstrating that PPB, spindle and phragmoplast orientation were defective in epidermal cells of both sab-5- and sab kuq -mutant root meristems ( Fig. 6e–q ; Supplementary Fig. S3f–h ). PPB, spindle and phragmoplast orientation in the sab-5;clasp-1 double mutant did not statistically differ from the sab-5 single mutant, but were significantly more strongly affected than in the clasp-1 single mutant ( Fig. 6o–q ). Thus, SAB function is required for cell division plane orientation already before or at the level of PPB orientation and sab shows epistasis over clasp during this process. Further, in comparison with wild type ( Fig. 6r ), the orientation of functional GFP-CLASP [21] on sab-5 mutant PPBs was affected and coincided with the misoriented alignment of PPB microtubules ( Fig. 6s,t ). These results suggested that SAB function is required for orientation of CLASP-guided cortical microtubules and stabilizes correct placement of PPB microtubules in the future plane of cell division. 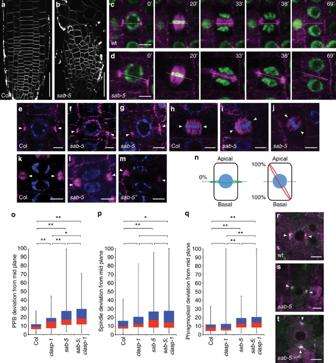Figure 6:sabis epistatic toclaspat mediating plane orientation. (a,b) Cell division orientation in root meristematic cells of 5-day-old (a) Col and (b)sab-5seedlings. Cells are outlined by FM4-64 fluorescence. (c,d) Live imaging of microtubules (mCherry-TUA5, magenta) and DNA (H2B-YFP, green) during cell division in meristems of 5-day-old seedlings. (c) Wild-type (wt;SAB/SABorSAB/sab-5), (d)sab-5homozygote (sab-5) cells. Number of cell division experiments analysed: wt,n=8;sab-5, n=7. Time points from preprophase band-(PPB)-marked prophase (0′) until the end of cytokinesis (69′) are indicated. Dotted lines, mitotic microtubule array or cell division orientation. (e–m) Mitotic microtubule array orientation in root meristematic cells are revealed by anti-α-tubulin immunolocalization (magenta). DAPI-labelled DNA, blue. (e–g) PPB in (e) wild type Col and (f,g)sab-5. (h–j) Metaphase plate in (h) Col and (i,j)sab-5. (k–m) Late phragmoplast in (k) Col and (l,m)sab-5.Angles of microtubule array orientation were obtained fromn=60 cells per mitotic stage, per genotype Col,clasp-1,sab-5andsab-5;clasp-1. Images forclasp-1andsab-5;clasp-1are not shown. (e–m) Arrowheads, plane of mitotic microtubule array orientation. (n) Microtubule array deviation from midplane are indicated as 0% (left) and 100% (right). (o–q) Quantitative, statistical analyses of anti-α-tubulin immunolocalization. (o) PPB, (p) metaphase plate, (q) late phragmoplast orientation in Col,clasp-1,sab-5andsab-5;clasp-1. (o–q) Box-and-whiskers plots forn=60 cells per mitotic stage, per genotype. Whiskers, maximum and minimum values of population. Blue boxes, 25% of values above median. Red boxes, 25% of values below median. Statistical differences between populations determined by K–S test are indicated as *P<0.05 and **P<0.01 (significance levelP<0.05). For exactP-values, seeSupplementary Table S2. Note,sab-5;clasp-1does not significantly differ fromsab-5ino–q, but significantly differs from Col andclasp-1inoandq. (r–t) Orientation (arrowheads) and co-localization (white) of GFP-CLASP (green) with mCherry-TUA5 (magenta) at PPBs of (r) wild-type (wt;SAB/SABorSAB/sab-5) and (s,t)sab-5homozygotes (sab-5). (s,t) Note, aberrant PPB orientation insab-5. Scale bars, 50 μm (a,b), 5 μm (c–m,r–t). Figure 6: sab is epistatic to clasp at mediating plane orientation. ( a , b ) Cell division orientation in root meristematic cells of 5-day-old ( a ) Col and ( b ) sab-5 seedlings. Cells are outlined by FM4-64 fluorescence. ( c , d ) Live imaging of microtubules (mCherry-TUA5, magenta) and DNA (H2B-YFP, green) during cell division in meristems of 5-day-old seedlings. ( c ) Wild-type (wt; SAB/SAB or SAB/sab-5 ), ( d ) sab-5 homozygote ( sab-5 ) cells. Number of cell division experiments analysed: wt, n =8; sab-5, n =7. Time points from preprophase band-(PPB)-marked prophase (0′) until the end of cytokinesis (69′) are indicated. Dotted lines, mitotic microtubule array or cell division orientation. ( e – m ) Mitotic microtubule array orientation in root meristematic cells are revealed by anti-α-tubulin immunolocalization (magenta). DAPI-labelled DNA, blue. ( e – g ) PPB in ( e ) wild type Col and ( f , g ) sab-5 . ( h – j ) Metaphase plate in ( h ) Col and ( i , j ) sab-5 . ( k – m ) Late phragmoplast in ( k ) Col and ( l , m ) sab-5. Angles of microtubule array orientation were obtained from n =60 cells per mitotic stage, per genotype Col, clasp-1 , sab-5 and sab-5;clasp-1 . Images for clasp-1 and sab-5;clasp-1 are not shown. ( e – m ) Arrowheads, plane of mitotic microtubule array orientation. ( n ) Microtubule array deviation from midplane are indicated as 0% (left) and 100% (right). ( o – q ) Quantitative, statistical analyses of anti-α-tubulin immunolocalization. ( o ) PPB, ( p ) metaphase plate, ( q ) late phragmoplast orientation in Col, clasp-1 , sab-5 and sab-5;clasp-1 . ( o – q ) Box-and-whiskers plots for n =60 cells per mitotic stage, per genotype. Whiskers, maximum and minimum values of population. Blue boxes, 25% of values above median. Red boxes, 25% of values below median. Statistical differences between populations determined by K–S test are indicated as * P <0.05 and ** P <0.01 (significance level P <0.05). For exact P -values, see Supplementary Table S2 . Note, sab-5;clasp-1 does not significantly differ from sab-5 in o – q , but significantly differs from Col and clasp-1 in o and q . ( r – t ) Orientation (arrowheads) and co-localization (white) of GFP-CLASP (green) with mCherry-TUA5 (magenta) at PPBs of ( r ) wild-type (wt; SAB/SAB or SAB/sab-5 ) and ( s , t ) sab-5 homozygotes ( sab-5 ). ( s , t ) Note, aberrant PPB orientation in sab-5 . Scale bars, 50 μm ( a , b ), 5 μm ( c – m , r – t ). Full size image SAB acts on cortical microtubule arrays We next analysed potential effects of SAB on cortical microtubule orientation in late meristematic epidermal cells at the transition to cell elongation, in rapidly expanding cells, and during later stages of hair cell differentiation. Strikingly, in contrast to the transversal orientation of mCherry-TUA5-marked microtubules observed in both late meristematic cells ( Supplementary Fig. S4a ) and in rapidly elongating wild-type cells ( Fig. 7a ), sab-5 -mutant cells of the same size displayed a more random orientation of cortical microtubules than wild-type cells in both cases ( Supplementary Fig. S4b,c ; Fig. 7b,c ). We further monitored the directionality of microtubule growth using the microtubule plus end-tracking protein (+TIP) AtEB1a-GFP [35] in combination with mCherry-TUA5. This revealed bidirectional movement of transversally oriented cortical microtubules in elongating wild-type cells and of the more randomly oriented microtubules in sab-5 -mutant epidermal cells ( Fig. 7a,b ; Supplementary Movies 3 and 4 ). Intriguingly, elongating trichoblasts just before hair initiation displayed a reoriented, bipolar arrangement of longitudinally growing microtubules ( Fig. 7d ; Supplementary Movie 5 ), where the majority of microtubule plus ends grew with apical directionality at apical ends of cells ( Fig. 7e ) and with basal directionality at basal ends of cells ( Fig. 7f ). This bipolarity of microtubule growth resembled the one recently described for elongating hypocotyl cells [36] . The overall longitudinal orientation and bipolarity of microtubule growth was less clearly axially aligned in sab-5 -mutant cells ( Fig. 7g ; Supplementary Movie 6 ). In addition, mCherry-TUA5 co-visualized with the root hair initiation site marker PIP5K3-YFP [37] revealed an accumulation of radially reorganized cortical microtubules at the root hair initiation site in 45% of the cells observed (32/71; Fig. 7h–l ; Supplementary Fig. S4d,e ), whereas 55% did not harbour such an array ( Supplementary Fig. S4f,g ). The majority of cells (94%, 67/71) at this differentiation stage showed longitudinally oriented microtubules interspersed in diffuse, cytosolic mCherry-TUA5 fluorescence indicative of microtubule depolymerization and reorganization in these cells ( Fig. 7i ; Supplementary Fig. S4d–g ). In comparison, only a minority of cells (6%, 4/71) still revealed transversal microtubule orientation, when hair initiation sites were already marked by PIP5K3-YFP. Although we did occasionally observe reorganized cortical microtubules at PIP5K3-YFP-marked hair initiation sites in sab-5- mutant cells ( Fig. 7m–o ), none of these cells (0%, 0/50) displayed one unique radial rearrangement that could be unambiguously identified as preceding a hair initiation site comparable to the situation in wild type ( Fig. 7m–o ; Supplementary Fig. S4h–k ). Hence, because of the irregular cortical microtubule arrangement in sab-5 , microtubule organization did not allow for prediction of the positions of hair initiation sites. However, PIP5K3-YFP-marked hair initiation sites occurred in ectopic basal-most, or more apical positions along sab-5 -mutant hair cells ( Fig. 7m–p ; Supplementary Fig. S4h–k ), when compared with the wild type ( Fig. 7h–j,p ; Supplementary Fig. S4d–g ). These findings suggest that SAB activity is required for cortical microtubule reorganization at correct sites before hair outgrowth. Thus, SAB function mediates transversal microtubule alignment in elongating cells and polar placement of domains of reorganizing microtubules in cells initiating hair formation. 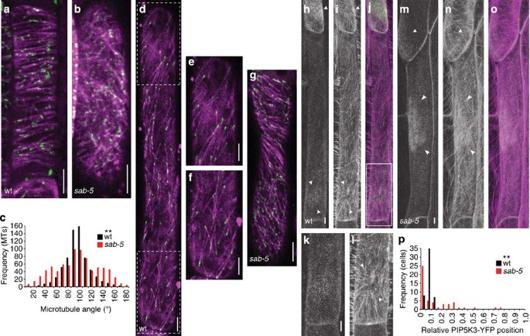Figure 7:SABis required for cortical microtubule orientation during cell elongation and planar polarity. (a,b) Live imaging of cortical microtubule arrays in early elongation stage root hair cells co-expressing mCherry-TUA5 (magenta) and the plus end-tracking protein AtEB1a-GFP (green). Note, (a) transversal orientation in wild type (wt;SAB/SABorSAB/sab-5), versus (b) more random orientation insab-5homozygote (sab-5). (c) Quantitative analysis of microtubule angles relative to the apical-basal cell axis in hair cells of 26–36 μm length from phenotypically wt andsab-5seedlings. Statistical analysis reveals highly significant difference between wt andsab-5(**P=0.000 by K–S test,n=673 microtubules analysed for wt andn=802 forsab-5, from 28 and 20 cells). For similar results on late meristematic cells of 13–18 μm length, seeSupplementary Fig. S4a–c. (d–g) Live imaging of cortical microtubule arrays in later elongation stage root hair cells co-expressing mCherry-TUA5 (magenta) and the plus end-tracking protein AtEB1a-GFP (green). (d) Bipolar axial orientation of microtubule growth in wt cell just before first hair formation. (e,f) Magnifications of regions marked ind, showing plus ends of microtubules preferentially growing towards (e) apical and (f) basal ends of cell. (g) Perturbed axial alignment and growth of microtubules insab-5-mutant cell. (h–o) Live co-imaging of mCherry-TUA5-labelled microtubules with hair initiation site marker PIP5K3-YFP. (h) PIP5K3-YFP, (i) mCherry-TUA5, (j) merge of PIP5K3-YFP (green) and mCherry-TUA5 (magenta) in wt cells. (k,l) Magnifications of inset inj,showing (k) PIP5K3-YFP and (l) mCherry-TUA5 at hair initiation site. (m) PIP5K3-YFP, (n) mCherry-TUA5, (o) merge of PIP5K3-YFP (green) and mCherry-TUA5 (magenta) insab-5. Arrowheads, microtubule (re-)organization at (i) close-to-basal site in wt versus (n) basal-most or apically shifted sites insab-5. (p) Quantitative analysis of polar PIP5K3-YFP patch position, marking site of root hair initiation. Number of cells in classes (frequency) showing PIP5K3-YFP position between basal (0) and apical (1) ends of epidermal cells is shown (**P=0.000 wt versussab-5by K–S test,n=50 cells per genotype from 39 wt and 41sab-5roots). For additional microtubule visualization, seeSupplementary Fig. S4d–k. Scale bars, 5 μm. Figure 7: SAB is required for cortical microtubule orientation during cell elongation and planar polarity. ( a , b ) Live imaging of cortical microtubule arrays in early elongation stage root hair cells co-expressing mCherry-TUA5 (magenta) and the plus end-tracking protein AtEB1a-GFP (green). Note, ( a ) transversal orientation in wild type (wt; SAB/SAB or SAB/sab-5 ), versus ( b ) more random orientation in sab-5 homozygote ( sab-5 ). ( c ) Quantitative analysis of microtubule angles relative to the apical-basal cell axis in hair cells of 26–36 μm length from phenotypically wt and sab-5 seedlings. Statistical analysis reveals highly significant difference between wt and sab-5 (** P =0.000 by K–S test, n =673 microtubules analysed for wt and n =802 for sab-5 , from 28 and 20 cells). For similar results on late meristematic cells of 13–18 μm length, see Supplementary Fig. S4a–c . ( d – g ) Live imaging of cortical microtubule arrays in later elongation stage root hair cells co-expressing mCherry-TUA5 (magenta) and the plus end-tracking protein AtEB1a-GFP (green). ( d ) Bipolar axial orientation of microtubule growth in wt cell just before first hair formation. ( e , f ) Magnifications of regions marked in d , showing plus ends of microtubules preferentially growing towards ( e ) apical and ( f ) basal ends of cell. ( g ) Perturbed axial alignment and growth of microtubules in sab-5 -mutant cell. ( h – o ) Live co-imaging of mCherry-TUA5-labelled microtubules with hair initiation site marker PIP5K3-YFP. ( h ) PIP5K3-YFP, ( i ) mCherry-TUA5, ( j ) merge of PIP5K3-YFP (green) and mCherry-TUA5 (magenta) in wt cells. ( k , l ) Magnifications of inset in j, showing ( k ) PIP5K3-YFP and ( l ) mCherry-TUA5 at hair initiation site. ( m ) PIP5K3-YFP, ( n ) mCherry-TUA5, ( o ) merge of PIP5K3-YFP (green) and mCherry-TUA5 (magenta) in sab-5 . Arrowheads, microtubule (re-)organization at ( i ) close-to-basal site in wt versus ( n ) basal-most or apically shifted sites in sab-5 . ( p ) Quantitative analysis of polar PIP5K3-YFP patch position, marking site of root hair initiation. Number of cells in classes (frequency) showing PIP5K3-YFP position between basal (0) and apical (1) ends of epidermal cells is shown (** P =0.000 wt versus sab-5 by K–S test, n =50 cells per genotype from 39 wt and 41 sab-5 roots). For additional microtubule visualization, see Supplementary Fig. S4d–k . Scale bars, 5 μm. Full size image SAB subcellular localization We next determined the subcellular localization of the predicted full-length 290 kDa SAB protein encoded by a messenger RNA of low abundance [27] , [28] . To this end, we employed recombineering [38] to insert three consecutive copies of the cDNA encoding for the bright fluorescent protein Ypet (3xYpet) at the 5′- or at the 3′-end of the genomic coding sequence of SAB. Both constructs rescued the overall sab-5 growth defect and all phenotypes investigated, including cell division plane orientation and planar polarity of root hair initiation ( Fig. 8a–g ). The planar polarity phenotype of sab-5 was fully rescued by SAB-3xYpet and largely, albeit not completely, by 3xYpet-SAB ( Fig. 8f,g ). Both constructs were expressed at low levels throughout the root tip and displayed indistinguishable subcellular distribution ( Figs 8h–l and 9a,b ). These results suggested a likely orientation of both the N- and the C-terminus towards the cytosol because fluorescence of cell wall-oriented GFP and YFP protein tags has been reported to be quenched by the low cell wall pH (refs 39 , 40 ). 3xYpet-SAB and SAB-3xYpet localized in patches at the cell periphery, suggesting localization to the plasma membrane or cell wall and to endomembrane compartments ( Figs 8k,l and Fig. 9a,b ). Plasmolysis experiments in the presence of a cell wall marker revealed retraction of SAB-3xYpet from the cell wall ( Fig. 9c,d ). Strikingly, meristematic cells showed clear enrichment of SAB-3xYpet at domains of apical and basal plasma membranes that had just started to retract from the cell wall at the onset of plasmolysis ( Fig. 9c ). Similarly, transversal, apical-basal membranes of non-plasmolysed cells showed an enrichment of SAB-3xYpet ( Fig. 9a ) and 3xYpet-SAB co-localization with the plasma membrane marker NSPN12-mCherry/WAVE131R (ref. 41 ; Fig. 9e ). Co-visualization of SAB-3xYpet with endoplasmic reticulum (ER; Fig. 9f ), Golgi ( Fig. 9g ) and trans -Golgi network (TGN) ( Fig. 9h ) markers [41] , [42] revealed that the endomembrane compartments containing 3xYpet-SAB/SAB-3xYpet did neither represent ER, Golgi nor TGN ( Fig. 9f–h ). Our findings do not support the previously posed hypotheses that full-length SAB-like proteins may be Golgi-localized or secreted at steady state, respectively [28] , [30] . Rather, our results provide in vivo evidence corroborating the identification of SAB peptides from plasma membrane preparations by proteomic approaches [43] . Further, SAB-3xYpet accumulated in small patches at the nuclear envelope where it co-labelled with microtubules marked by mCherry-TUA5 during mitotic prophase ( Fig. 9i ). At the cell cortex, SAB-3xYpet did not precisely co-localize with PPB microtubules but consistently closely associated with them in the majority of prophase cells analysed (91%, 84/92) ( Fig. 9i , arrowheads; Supplementary Fig. S5a–f ). Strikingly, SAB-3xYpet was also found in patches along mitotic spindle microtubules ( Fig. 9j,k ), located to cell plate membranes from early to late stages of cell plate formation ( Fig. 9l–n ), and subsequently remained at domains of apical and basal membranes of dividing cells ( Fig. 9e,n ). These findings were confirmed in co-labelling studies with rhodamine phalloidin for F-actin staining in aldehyde-fixed cells ( Fig. 9o–t ) and by co-labelling of the KNOLLE cell plate syntaxin with SAB-3xYpet at the cell plate ( Fig. 9u ). In elongating epidermal cells, SAB-3xYpet distributed more evenly in endomembrane compartments of unknown identity throughout the cytosol ( Fig. 9b ). In more differentiated cells, where SAB-3xYpet expression was very low and just detectable above background, SAB-3xYpet compartments were present, although not much enriched, at sites of root hair initiation before morphological outgrowth ( Fig. 9v,w ). Taken together, we show that SAB localizes to plasma membrane domains, preferentially but not exclusively to apical and basal plasma membranes of meristematic cells, at the nuclear periphery, flanking the PPB at the onset of mitosis, to mitotic spindles, to cell plate membranes as well as to as yet unidentified endomembrane compartments. Thus, SAB is present in most root tip cells including dividing, elongating and differentiating epidermal cells, consistent with its functions in epidermal cells reported here. 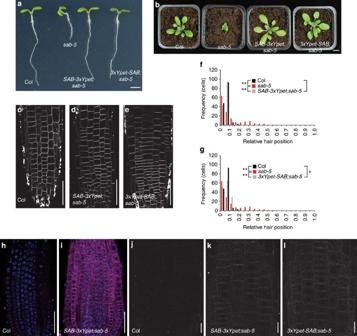Figure 8: SAB-3xYpet and 3xYpet-SAB rescuesab-5phenotypes and display identical localization. (a) Five-day-old seedlings, (b) 21-day-old plants of Col,sab-5,SAB-3xYpet;sab-5and3xYpet-SAB;sab-5. Note, rescue ofsab-5growth defects. (c–e) Cell division orientation in root meristem of 5-day-old (c) Col, (d)SAB-3xYpet;sab-5and (e)3xYpet-SAB;sab-5seedlings. Cells outlined by FM4-64 fluorescence. (f,g) Quantitative analysis of planar polarity in (f)SAB-3xYpet;sab-5and (g)3xYpet-SAB;sab-5compared with Col andsab-5is displayed as relative root hair position similar toFig. 1c. **P=0.000 Col versussab-5;P=0.422 Col versusSAB-3xYpet;sab-5; **P=0.000sab-5versusSAB-3xYpet;sab-5; *P=0.019 Col versus3xYpet-SAB;sab-5; **P=0.000sab-5versus3xYpet-SAB;sab-5by K–S test,n=150 cells from 30 roots per genotype. Note, (f) full rescue ofsab-5planar polarity defects by SAB-3xYpet and (g) partial rescue by 3xYpet-SAB. (h,i) Expression of SAB-3xYpet throughout the root meristem was detected by immunolabelling with anti-GFP antibody (magenta), DAPI (blue), of (h) Col and (i)SAB-3xYpet;sab-5seedlings. Images are transversal sections showing SAB-3xYpet signal in all cell layers. (j–l) Live imaging of (j) Col, (k)SAB-3xYpet;sab-5and (l)3xYpet-SAB;sab-5seedlings showing indistinguishable subcellular localization of SAB-3xYpet and 3xYpet-SAB in root meristematic epidermal cells. Scale bars, 2 mm (a), 10 mm (b), 50 μm (c–e,h,i), 10 μm (j–l). Figure 8: SAB-3xYpet and 3xYpet-SAB rescue sab-5 phenotypes and display identical localization. ( a ) Five-day-old seedlings, ( b ) 21-day-old plants of Col, sab-5 , SAB-3xYpet ; sab-5 and 3xYpet-SAB;sab-5 . Note, rescue of sab-5 growth defects. ( c – e ) Cell division orientation in root meristem of 5-day-old ( c ) Col, ( d ) SAB-3xYpet;sab-5 and ( e ) 3xYpet-SAB ; sab-5 seedlings. Cells outlined by FM4-64 fluorescence. ( f , g ) Quantitative analysis of planar polarity in ( f ) SAB-3xYpet ; sab-5 and ( g ) 3xYpet-SAB;sab-5 compared with Col and sab-5 is displayed as relative root hair position similar to Fig. 1c . ** P =0.000 Col versus sab- 5; P =0.422 Col versus SAB-3xYpet ; sab-5 ; ** P =0.000 sab-5 versus SAB-3xYpet ; sab-5 ; * P =0.019 Col versus 3xYpet-SAB ; sab-5 ; ** P =0.000 sab-5 versus 3xYpet-SAB ; sab-5 by K–S test, n =150 cells from 30 roots per genotype. Note, ( f ) full rescue of sab-5 planar polarity defects by SAB-3xYpet and ( g ) partial rescue by 3xYpet-SAB. ( h , i ) Expression of SAB-3xYpet throughout the root meristem was detected by immunolabelling with anti-GFP antibody (magenta), DAPI (blue), of ( h ) Col and ( i ) SAB-3xYpet;sab-5 seedlings. Images are transversal sections showing SAB-3xYpet signal in all cell layers. ( j – l ) Live imaging of ( j ) Col, ( k ) SAB-3xYpet ; sab-5 and ( l ) 3xYpet-SAB ; sab-5 seedlings showing indistinguishable subcellular localization of SAB-3xYpet and 3xYpet-SAB in root meristematic epidermal cells. Scale bars, 2 mm ( a ), 10 mm ( b ), 50 μm ( c – e , h , i ), 10 μm ( j – l ). 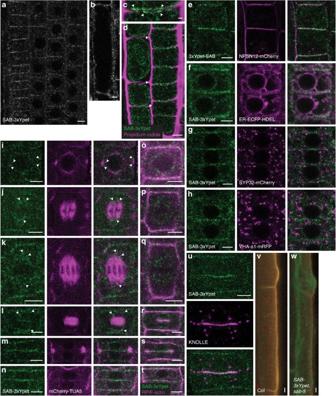Figure 9: SAB subcellular localization. (a–h,v,w) Live imaging of functional SAB-3xYpet or 3xYpet-SAB in root epidermal cells of 5-day-old seedlings. (a,b) SAB-3xYpet insab-5background detected in (a) meristematic cells and (b) elongating cells. (c,d) Onset of plasmolysis in 5-day-old,SAB-3xYpet;sab-5seedling root co-labelled for SAB-3xYpet (green) and cell wall stain propidium iodide (magenta). Note, (c) apical and basal membrane domain labelling (arrowheads) and (d) separation of SAB-3xYpet from cell wall (arrowheads). (e–h) Meristematic root epidermal cells. (e) 3xYpet-SAB (green) co-localizes with plasma membrane marker NPSN12-mCherry/WAVE131R (magenta). (f–h) SAB-3xYpet (green) co-detected with (f) ER marker ER-ECFP-HDEL (magenta), (g) Golgi marker SYP32-mCherry/WAVE22R (magenta) and (h) TGN marker VHA-a1-mRFP (magenta). Merged channels to the right ine–h. Note, (f) little co-localization and (g,h) no co-localization when compared withe. (i–t) SAB-3xYpet (green) (i–n) co-expressed with mCherry-TUA5 (magenta) and (o–t) co-labelled with rhodamine phalloidin (magenta) for F-actin visualization (RP/F-actin) in paraformaldehyde-fixed roots. (i) Prophase. SAB-3xYpet and mCherry-TUA5 fluorescence around the nuclear envelope. Note, association of SAB-3xYpet (arrowheads) with PPB but no direct co-localization (see alsoSupplementary Fig. S5). (o) Late prophase. SAB-3xYpet and RP/F-actin. (j,k) SAB-3xYpet localization at mitotic spindles preferentially towards the periphery (arrowheads) in (j,p) metaphase and (k,q) anaphase. (l,r) Late telophase. (l) SAB-3xYpet in centre of phragmoplast at early cell plate and at remaining spindle microtubules (arrowheads). (r) SAB-3xYpet co-labelling with F-actin at early cell plate. (m,s) Late cytokinesis. SAB-3xYpet at cell plate co-labelling with (m) peripheral phragmoplast microtubules and (s) peripheral phragmoplast F-actin. (n,t) End of cytokinesis. SAB-3xYpet at transversal (apical, basal) plasma membranes. (u) anti-KNOLLE cell plate marker immunofluorescence (magenta) and SAB-3xYpet (green) fluorescence. Channel merge (lower panel) indicates co-localization at cell plate. (v,w) Elongated epidermal cells undergoing hair initiation and bulge outgrowth, visualized by colour-coded spectral lambda scan between 416 and 686 nm. Ypet-specific fluorescence, green. (v) Wild type Col. (w) GenomicSAB-3xYpet;sab-5. Images ina–wacquired with LSM780 32-channel gallium arsenide phosphide detector array. Scale bars, 5 μm (a,b,d–x), 1 μm (c). Full size image Figure 9: SAB subcellular localization. ( a – h , v , w ) Live imaging of functional SAB-3xYpet or 3xYpet-SAB in root epidermal cells of 5-day-old seedlings. ( a , b ) SAB-3xYpet in sab-5 background detected in ( a ) meristematic cells and ( b ) elongating cells. ( c , d ) Onset of plasmolysis in 5-day-old, SAB-3xYpet ; sab-5 seedling root co-labelled for SAB-3xYpet (green) and cell wall stain propidium iodide (magenta). Note, ( c ) apical and basal membrane domain labelling (arrowheads) and ( d ) separation of SAB-3xYpet from cell wall (arrowheads). ( e – h ) Meristematic root epidermal cells. ( e ) 3xYpet-SAB (green) co-localizes with plasma membrane marker NPSN12-mCherry/WAVE131R (magenta). ( f – h ) SAB-3xYpet (green) co-detected with ( f ) ER marker ER-ECFP-HDEL (magenta), ( g ) Golgi marker SYP32-mCherry/WAVE22R (magenta) and ( h ) TGN marker VHA-a1-mRFP (magenta). Merged channels to the right in e – h . Note, ( f ) little co-localization and ( g , h ) no co-localization when compared with e . ( i – t ) SAB-3xYpet (green) ( i – n ) co-expressed with mCherry-TUA5 (magenta) and ( o – t ) co-labelled with rhodamine phalloidin (magenta) for F-actin visualization (RP/F-actin) in paraformaldehyde-fixed roots. ( i ) Prophase. SAB-3xYpet and mCherry-TUA5 fluorescence around the nuclear envelope. Note, association of SAB-3xYpet (arrowheads) with PPB but no direct co-localization (see also Supplementary Fig. S5 ). ( o ) Late prophase. SAB-3xYpet and RP/F-actin. ( j , k ) SAB-3xYpet localization at mitotic spindles preferentially towards the periphery (arrowheads) in ( j , p ) metaphase and ( k , q ) anaphase. ( l , r ) Late telophase. ( l ) SAB-3xYpet in centre of phragmoplast at early cell plate and at remaining spindle microtubules (arrowheads). ( r ) SAB-3xYpet co-labelling with F-actin at early cell plate. ( m , s ) Late cytokinesis. SAB-3xYpet at cell plate co-labelling with ( m ) peripheral phragmoplast microtubules and ( s ) peripheral phragmoplast F-actin. ( n , t ) End of cytokinesis. SAB-3xYpet at transversal (apical, basal) plasma membranes. ( u ) anti-KNOLLE cell plate marker immunofluorescence (magenta) and SAB-3xYpet (green) fluorescence. Channel merge (lower panel) indicates co-localization at cell plate. ( v , w ) Elongated epidermal cells undergoing hair initiation and bulge outgrowth, visualized by colour-coded spectral lambda scan between 416 and 686 nm. Ypet-specific fluorescence, green. ( v ) Wild type Col. ( w ) Genomic SAB-3xYpet ; sab-5 . Images in a – w acquired with LSM780 32-channel gallium arsenide phosphide detector array. Scale bars, 5 μm ( a , b , d – x ), 1 μm ( c ). Full size image Our study unravels new roles for the large SAB protein related to uncharacterized proteins found throughout eukaryotes. We report important functions for SAB in PPB, spindle, phragmoplast and cell division plane orientation, cortical microtubule orientation and planar polarity establishment. Moreover, we uncover biological functions of SAB in cell and planar polarity that it shares with CLASP . A role for CLASP function during microtubule-dependent PIN2 polarity establishment in cortical cells and PIN2 abundance modulated by endocytosis has recently attracted attention [18] , [19] . Although SAB and CLASP do not appreciably affect apical epidermal PIN2 polarity, we uncover that CLASP mediates establishment of planar polarity of ROP and root hair positioning, and we confirm a previously reported role of CLASP in PPB orientation [15] , [16] . Intriguingly, however, our results unravel that sab mutations perturb all investigated processes more strongly than clasp mutations. sab affects PPB, spindle and phragmoplast orientation as well as planar root hair polarity more strongly than clasp , and shows an epistatic interaction with clasp . Synergistic action of SAB and CLASP in controlling root length and trichome branching may reflect additional nonlinear interaction, including potential feedback regulation. Alternatively, synergistic action can be interpreted by interaction of SAB and CLASP with additional partners during these two processes. However, during PPB, spindle and phragmoplast orientation as well as planar polarity in root epidermal cells, SAB and CLASP act sequentially. Moreover, SAB likely acts upstream of CLASP considering the misorientation of CLASP-labelled PPBs observed in sab, the stronger phenotypes of sab mutants and the epistatic relationship of sab over clasp . Hence, our observations mechanistically link SAB function to CLASP-guided cortical microtubule organization during these processes. We further describe a newly observed bipolar arrangement of longitudinally growing microtubules at later stages of root hair cell elongation. Although striking and similar to the bipolar arrangement recently observed in hypocotyl cells [36] , the functional importance of this dynamic bipolar reorganization, and how it may affect polar site selection during root hair initiation, remains to be determined. Further, we find that sab is epistatic to clasp during polar placement of ROP protein patches at sites of hair initiation where we observe cortical microtubule reorganization before morphological onset of hair outgrowth. Earlier observations have implicated microtubules in tip growth of different cell types in various organisms [14] , [44] , [45] , [46] , and radial microtubule alignment has been observed, for example, in tips of moss protonemata [44] as well as in conifer pollen tubes [45] . In addition, microtubule dynamics are known to have a function in directing the growth of and limiting the number of growth sites in root hairs [46] , [47] . Our work also points out a role for microtubule reorganization in polarity of root hair cells. However, we report that microtubules are involved earlier than previously described, namely, during selection of the site of root hair initiation. This suggests that the microtubule cytoskeleton acts both in determining planar polarity of hair cell differentiation and in maintaining polar tip growth of root hairs. It remains to be determined how SAB affects microtubule reorganization at the molecular level because the genetic interactions observed between SAB and CLASP may not necessarily reflect direct interaction at the protein level. Yet, SAB-3xYpet localized to the perinuclear region from where microtubules radiate towards the PPB as well as adjacent to the PPB, suggesting that SAB may be, directly or indirectly, involved in nucleation or guidance of PPB microtubules. This localization does, however, not match exactly the distribution of CLASP, which directly co-localizes with PPB microtubules at cell edges and binds to microtubule plus ends [20] , [21] . This suggests that the observed genetic interactions may reflect an indirect or transient interaction within the same pathway. The SAB protein localizes to spindle microtubules from early prophase, and later on is observed close to the spindle periphery consistent with our findings that SAB is required for spindle and phragmoplast orientation. Further, the accumulation of SAB at cell plate membranes in the centre of the phragmoplast and on apical and basal plasma membranes opens the door for future studies on the role of SAB at these sites. Hence, our work paves the way to elucidating the molecular function of SAB in microtubule reorganization during cell division plane orientation, cell and planar polarity formation in plants. It also encourages further studies on the connection between SAB-related proteins and the microtubule cytoskeleton. Future studies may now address what proteins the large membrane protein SAB interacts with at the molecular level and which of the homology regions observed in SAB-like proteins throughout eukaryotes may be required for such interactions. Interestingly, the human genome encodes a single SAB-related predicted 2,235 amino-acid-long protein of unknown function named KIAA0100, which is overexpressed in human cancers and also known as, for example, breast cancer overexpressed1 or monocytic leukaemia-associated antigen22 (refs 48 , 49 , 50 , 51 ). Hence, our findings linking SAB to CLASP-mediated microtubule organization may provide a stepping stone for functional analysis of SAB-related proteins during eukaryotic development and for dissecting their potential role in human cancer. Plant growth conditions Medium and growth conditions were as described [4] . In brief, seeds were surface sterilized and stratified at 4 °C for 3 days before plating on MS plates (1 × MS medium, 1% sucrose, 0.8% plant agar, 1 M morpholinoethanesulphonic acid, pH 5.7). Seedlings were grown vertically at 23 °C day and 18 °C night under 16 h light/8 h dark photoperiod and subjected to analysis after 5 days. Plant material and genotyping Arabidopsis thaliana ecotype Columbia (Col-0) was employed as a wild type and as background for the kuq mutant; the following T-DNA insertion lines from the SALK collection [52] were obtained from the Nottingham Arabidopsis Stock Centre: sab-5 (stock number N608709), sab-6 (N552995), sab-7 (N623771) and sab-8 (N512897). All above sab alleles, with the exception of sab-7 , were unable to self-fertilize and produced 5–10 seeds per silique on pollination with wild-type pollen. Lines were maintained as heterozygotes and molecular genotyping was used to identify plants carrying mutant alleles. Other previously described mutants and transgenic lines were provided by the Nottingham Arabidopsis Stock Centre or corresponding authors of the cited publications: pPEN3:PEN3-GFP [53] , p35S:GFP-BASL [24] , clasp-1 (refs 15 , 16 ) (N620061), clasp-2 (refs 15 , 16 ) (N583034), p35S:mCherry-TUA5 (refs 32 , 33 ), p35S:H2B-YFP [34] , pCLASP:GFP-CLASP [21] , p35S:EB1a-GFP [35] , pGL2:NTF [54] , pPIP5K3:PIP5K3-YFP [37] , pUBQ10:NSPN12-mCherry/WAVE131R [41] , pUBQ10:SYP32-mCherry/WAVE22R [41] and VHA-a1-mRFP [42] . Other mutant and transgene combinations were generated in this study. Primers for PCR genotyping of mutants are listed in Supplementary Table S3 . Immunofluorescence and CLSM Whole-mount immunolabelling of roots was performed as described [4] . Antibody dilutions were the following: rabbit anti-ROP 1:25 (ref. 8 ); rabbit anti-PIN2 1:400 (ref. 55 ); mouse anti-α-tubulin DM1A 1:200 (Santa Cruz, Sc-32293); rabbit anti-GFP 1:1,000 (Torrey Pines, TP-401); rabbit anti-KNOLLE 1:4,000 (ref. 56 ); DY649 donkey anti-rabbit 1:800 (Jackson ImmunoResearch) for anti-ROP, anti-PIN2, anti-GFP; DyLight633 donkey anti-rabbit 1:100 (Agrisera, AS122034) for anti-KNOLLE; TRITC donkey anti-mouse 1:150 (Jackson ImmunoResearch). Donkey secondary antibodies for multilabelling pre-absorbed to crossreacting species were employed. DNA was stained with 4',6-diamidino-2-phenylindole (DAPI) (1 μg ml −1 , Sigma). Imaging of immunolabelled or live roots was carried out using either a Leica TCS SP2 AOBS (Leica) spectral confocal laser scanning microscopy (CLSM) system mounted on an Leica DM IRE2 inverted microscope or a Zeiss LSM780 spectral CLSM system equipped with a 32-channel gallium arsenide phosphide detector array and mounted on a Zeiss Axio observer Z1 inverted microscope. Laser excitation lines, emission filters and acquisition modes for all fluorophore combinations are listed in Supplementary Table S4 . Oil-corrected Plan-Apochromat 63 × objectives, numerical aperture 1.4 (HCX PL APO 63.0 × 1.40 OI BD UV, Leica; or DIC M27, Zeiss) were used for immunolabelling studies. For live imaging, a water-corrected C-Apochromat 40 × objective, numerical aperture 1.2 (M27, Zeiss) was used. It was not possible to detect 3xYpet-SAB and SAB-3xYpet fluorescent fusions with a Leica SP2 confocal microscope in live imaging studies because of extremely low intensity of the signal. Hence, all imaging of these lines was carried out with a Zeiss LSM780 microscope. It was however possible to detect SAB-3xYpet and 3xYpet-SAB with a Leica SP2 microscope after immunolabelling with anti-GFP antibody (Torrey Pines). Images were processed and analysed using ZEN2010 (Zeiss), ImageJ ( http://www.imagej.nih.gov/ij/ ) or Adobe Photoshop CS4 (Adobe Systems), and assembled in Adobe Illustrator CS3 (Adobe Systems). Analysis of root hair position and trichoblast length Quantitative microscopic analysis of root hair position and cell length was performed in three independent experiments as described [4] . Statistical analysis employed non-parametric Kolmogorov–Smirnov (K–S) test and two-tailed t -test. Quantitative analysis of ROP positioning Relative ROP position in trichoblasts before hair initiation was determined by immunolocalization as described [4] . Measurements were performed on n =50 cells per genotype, from 8 to 22 roots. Images were analysed using Leica Application Suite Advanced Fluorescence software (Leica). Scanning electron microscopy of leaf trichome orientation Growth of sab mutants was significantly slower compared with wild-type plants. To analyse leaves at a similar developmental stage, the third true leaf from 21-day-old sab plants was compared with the third true leaf from 14-day-old wild-type plants that did not obviously differ in trichome orientation from 21-day-old wild-type plants. Leaves were fixed in 2.5% glutaraldehyde in sodium cacodylate buffer overnight at room temperature. To keep the leaves submerged in the solution, the fixation was carried out in a desiccator with a low under-pressure to take away trapped air. Fixed material was dehydrated in increasing ethanol concentrations, up to pure ethanol, and was thereafter dried from liquid CO 2 using standard critical point drying technique (Polaron E3000 CPD apparatus, Quorum Technologies Ltd, Ashford, UK). Dried specimens were attached to specimen holders using adhesive carbon tape and thereafter coated with ~15 nm gold in an evaporation system. Microscopy was performed in a scanning electron microscope running at standard conditions (Carl Zeiss SMT/Cambridge Instruments 360iXP, Cambridge, UK) and micrographs were recorded at standardized magnifications and locations on the leaves. Trichome orientation was investigated in a rectangle of 2 mm × 1.5 mm in the centre of the leaf adaxial surface. Angles between the proximal-distal leaf axis and the trichome’s first branch were measured on scanning electron microscope images using ImageJ. Isolation and positional cloning of kuq The kuq mutant was isolated in a genetic screen of 5-day-old seedlings for aberrant planar polarity of root hair positioning. A population of ~20,000 M 2 seedlings obtained from ~2,500 fast-neutron-mutagenized M 1 plants (Col-0 ecotype, Lehle Seeds) were grown vertically and screened by stereomicroscopy. kuq was characterized by a more random root hair position along epidermal cells, shorter and radially swollen roots and bent cotyledons. The semi-sterile kuq mutant was fertilized with Col-0 pollen and produced five to eight seeds, which were subjected to further analyses. The kuq phenotype segregated at 27% ( n =496) after backcrossing, indicating that it was caused by a single, recessive mutation. kuq was crossed to Landsberg erecta (L er ) to generate a mapping population, and genomic DNA (gDNA) was extracted from 1,298 F 2 seedlings displaying the kuq phenotype and used for mapping by positional cloning [57] . SSLP and CAPS molecular markers were generated as described [57] and by using the Monsanto Arabidopsis Polymorphism Collection ( http://www.arabidopsis.org/browse/Cereon/index.jsp ), and the mutation was mapped to a 480-kb interval on chromosome 1 ( Fig. 2 ). Analysis of T-DNA insertion lines in genes within this interval suggested the SABRE ( SAB ) gene as the strongest candidate, with 9 T-DNA lines whose homozygous seedlings looked indistinguishable from kuq mutants. The entire ~14.5 kb SAB genomic region was PCR amplified from kuq mutants and sequenced with three times coverage. This revealed a single cytosine deletion in the 17th exon of the SAB gene, at position 6,592 (of 7,824) of the coding sequence. The mutation caused a frame shift that was calculated to introduce a stop codon at position 6,617–6,619, truncating the predicted SAB protein after amino acid 2,205 (of 2,607). A CAPS marker designed over the mutated site physically confirmed the nucleotide deletion and allowed molecular genotyping of kuq mutants (see Supplementary Table S3 ). RT–PCR analysis Total RNA was extracted from roots of 5-day-old seedlings employing the RNeasy Plant Mini Kit (Qiagen) according to manufacturer’s instructions. Two biological replicates were analysed for each mutant and the respective wild-type control. RNA was purified with the Ambion DNA-free Kit (Ambion), precipitated with LiCl and resuspended in diethyl pyrocarbonate-treated H 2 O. cDNA was synthesized using iScript cDNA Sythesis Kit (Bio-Rad) and used for semiquantitative RT–PCR analysis with primer pairs spanning the T-DNA insertion (or single-nucleotide deletion), and primer pairs located respectively at the 5′- and 3′-end of the SAB gene ( Supplementary Table S3 for primer sequences). Primer pairs were designed to span introns to identify potential gDNA contaminations. Primers amplifying the ELONGATION FACTOR 1-α ( EF1-α ) or ADENINE PHOSPHORIBOSYL TRANSFERASE 1 ( APT1 ) genes were used as controls. Reactions were carried out with 34 cycles for T-DNA insertion spanning primers (22 cycles for EF1-α primers) and 35 cycles for primers located close to the 5′- or 3′- end of the SAB gene (35 and 40 cycles for APT1 primers, respectively). Analysis of SAB evolutionary conservation Searches for proteins with similarity to SAB were performed with Blastp version 2.2.28+ ( http://www.blast.ncbi.nlm.nih.gov/blast/Blast.cgi ) with default parameters using full SAB sequence (At1g58250.1) against non-redundant protein sequences database. Alignment of Saccharomyces cerevisiae and Schizosaccharomyces pombe proteins was achieved after second PSI-BLAST iteration. Full sequences of SAB-related proteins from selected species were aligned with MUSCLE version 3.8.31 ( http://www.ebi.ac.uk/Tools/services/web/toolform.ebi?tool=muscle ). Output phenogramme generated from second iteration was visualized with Phylodendron Phylogenetic tree printer ( http://www.iubio.bio.indiana.edu/treeapp/treeprint-form.html ). Trichome branching analysis Measurements of trichome branching were performed as described [15] . Third true leaf of 21-day-old plants was observed with a Leica MZ 9.5 stereomicroscope (Leica), and number of branches was counted for all trichomes on adaxial leaf surface. Number of leaves (plants) analysed are as follows: 10 for Col-0, 12 for clasp-1 , 16 for sab kuq , 16 for sab-5 and 16 for sab-5;clasp-1 . FM4-64 staining Seedlings were incubated in 1 × MS medium with 25 μM FM4-64 (Molecular Probes) for 5 min on ice. After two washes with 1 × MS medium on ice, seedlings were mounted on cover slips in 1 × MS medium. Live imaging of microtubules and nuclei during cell division Wild-type looking and sab-5 seedlings expressing mCherry-TUA5 (ref. 32 ) and H2B-YFP [34] were imaged live. A region of 53.14 μm × 53.14 μm centred on a meristematic cell in prophase (displaying clear PPB) was visualized at intervals of 1 min throughout cell division. For each time point, Z stacks of six optical sections at 0.46 μm distance were acquired, and the image closest to the centre of the cell was selected. Imaging windows and planes were constantly adjusted to account for movement of roots in X-, Y - and Z -direction. Images of each time point were aligned using ImageJ Stackreg plugin ( http://www.bigwww.epfl.ch/thevenaz/stackreg/ ) before movie assembly. Analysis of mitotic figure orientation Seedlings were labelled with mouse anti-α-tubulin antibody (Santa Cruz). Z stacks were acquired from meristematic cells in prophase, metaphase and late cytokinesis, and images closest to the centre of the cell were selected. For each cell, length of the longitudinal cell edges and distances between the transversal cell edges and the points where the PPB ring or phragmoplast touched the longitudinal edges were measured. Deviation of PPB, mitotic spindle and phragmoplast orientation from the transversal central axis (midplane) of the cell was indicated by the absolute value derived by the following formula: 100−(distance between transversal edge and mitotic structure/total length of longitudinal edge × 200). A mean of 0% between the two values calculated for a cell (one corresponding to each side) indicated a structure passing through the midplane, whereas 100% was one tracing a diagonal of the cell. Higher deviations occurred rarely (2.5% of 720 cells in total) and were considered as 100% for further analysis. Box-and-whisker plots were used to visualize deviation from the midplane in the 60 cells examined for each genotype and mitotic stage: for each data set they display median, upper quartile (blue box), lower quartile (red box), maximum (upper whisker) and minimum (lower whisker) of the population. Live imaging of cortical microtubules Cortical microtubules were analysed in epidermal cells of seedlings expressing mCherry-TUA5 (ref. 32 ) and AtEB1a-GFP [35] or PIP5K3-YFP [37] . For movies of microtubule growth, Z stacks of planes intersecting the periclinal face of the cell 1 μm apart (0.51 μm in elongating wild-type cells) were imaged every 5 s for 2.5 min. Maximum intensity projections of each time point were used to assemble movies. For images of cortical microtubules in cells about to initiate outgrowth of a root hair, Z stacks of planes at 0.46 μm distance intersecting the periclinal face of the cell were acquired and employed to generate maximum intensity projections. Relative PIP5K3-YFP position was determined measuring the distance between basal trichoblast membrane and basal end of PIP5K3-YFP patch on the upper cell face and dividing it by total cell length. Measurements were performed on n =50 cells per genotype from 39 to 41 roots. Microtubule orientation measurements Seedlings with wild-type or sab-5 phenotype expressing the atrichoblast marker pGL2:NTF [54] and mCherry-TUA5 (ref. 32 ) were imaged live. Trichoblasts were identified by absence of pGL2:NTF. Z stacks of planes at 0.45 μm distance were acquired on the periclinal face from either meristematic cells of 13–18 μm or elongated cells of 26–36 μm cell length. Maximum intensity projections were used to measure the angle of microtubules with respect to the root growth axis. Generation of SAB-3xYpet and 3xYpet-SAB lines A 3xYpet tag was fused to SAB at either the C- or the N-terminus by recombineering [38] . The JAtY clone 63C14, purchased from the John Innes Centre (Norwich, UK), was selected based on bacterial artificial chromosome end sequence information from the Arabidopsis thaliana Integrated Database, http://www.atidb.org/cgi-perl/gbrowse/atibrowse/ . In this clone, the SAB-coding region is preceded and followed by 36 and 4.5 kb of gDNA, respectively. The JAtY transformation-competent bacterial artificial chromosome was transferred to Escherichia coli strain SW105, kindly provided by Dr N. Copeland (Mouse Cancer Genetics Program, National Cancer Institute Frederick, Frederick, MD, USA) [58] . A recombineering cassette was generated by inserting the ampicillin resistance gene flanked by flippase recognition sites at the 3′-end of the codon-optimized 3xYpet tag [38] (cassette available from the Arabidopsis Biological Resource Center, stock number CD3-1727). The cassette was amplified by PCR using two long recombineering primers ( Supplementary Table S3 ): the forward primer included 50 nucleotoides homologous to the region upstream of the 3xYpet insertion point (until right after the first codon of the SAB gene for the N-terminal fusion and before the STOP codon for the C-terminal fusion); the reverse primer included 50 nucleotides homologous to the region downstream of the insertion point (ending just after the first codon or before the STOP codon of SAB , respectively). Cassette recombination into the JAtY clone was performed as described [38] , and the Amp R marker was removed on induction of the Flippase gene expression by arabinose. Constructs were sequenced and respective transformation-competent bacterial artificial chromosome clones transformed into Agrobacterium tumefaciens GV3101, which was used to transform sab-5 heterozygous Arabidopsis plants by floral dipping [38] , [59] . Transformants were selected by Basta and further screened by PCR, ensuring presence of the sab-5 -mutant allele, of the tagged SAB gene, and of the SacB gene (for primer sequences Supplementary Table S3 ). SacB lies close to the T-DNA left border and its presence confirmed transfer of at least one full copy of the T-DNA to the plant genome [38] . T 2 seedlings were analysed for fluorescence using a Zeiss LSM780 confocal microscope. Out of 12 SAB-3xYpet lines analysed, 7 displayed a very weak but identical fluorescent signal. Out of 10 3xYpet-SAB lines, 9 showed the same pattern of fluorescence, indistinguishable from SAB-3xYpet lines. One line was selected for each construct and T 2 plants homozygous for the sab-5 allele and the SAB transgene were identified. Offspring of these plants was used for all further analyses and genetic crosses. Plasmolysis Plasmolysis was performed as described [60] . Seedlings were incubated in 1 ml of 0.8 M mannitol for 2 h under gentle agitation, stained for 30 s in 10 μg ml −1 propidium iodide in 0.8 M mannitol, mounted on cover slips in the same medium and immediately imaged. Generation of ER-ECFP-HDEL marker The binary vector pGreenII0229 (ref. 61 ; obtained from the John Innes Centre, Norwich) was modified by adding a Cauliflower mosaic virus 35S promoter (derived from the pSK36 vector [62] ) and a Nopaline synthase terminator between the Bam HI and Spe I, and at the Not I site of the multiple cloning site, respectively. The resulting vector was named p235S. ER signal peptide of Arabidopsis Basic chitinase (At3g12500) was amplified from gDNA using primers CHTTPFAscI and CHTTPRSpeI. PCR product was digested with Asc I and Spe I and cloned into the corresponding sites of the p235S vector, generating the p235S-TP construct. Enhanced cyan fluorescent protein (ECFP) coding sequence was amplified from the pECFP-C1 vector (Clontech) using primers CFPFSpeI and CFPERNotI, which introduced the coding sequence for the ER-retention signal peptide HDEL before the stop codon. PCR product was digested with Spe I and Not I and subcloned into the corresponding sites of the p235S-TP vector. After sequencing with 35SF and tNOSR primers, the resulting construct was transferred to A. tumefaciens strain C58C1 and used to transform Arabidopsis Col-0 plants by floral dipping [59] . T 1 transgenic plants were selected by Basta. Primer sequences are listed in Supplementary Table S3 . Visualization of SAB together with microtubules or F-actin Seedlings expressing SAB-3xYpet or SAB-3xYpet and mCherry-TUA5 were fixed for 40 min in PME buffer (50 mM piperazine-1,4-bis(2-ethanesulfonic acid), 2 mM MgSO 4 , 5 mM ethylene glycol-bis(β-aminoethylether)- N,N,N′,N′ -tetraacetic acid, pH 6.9) supplemented with 0.1% Triton X-100 and 2% paraformaldehyde as described [63] . After three washes with PME buffer, seedlings were either mounted on cover slips in PME buffer and immediately imaged (for seedlings expressing SAB-3xYpet and mCherry-TUA5) or, for visualization of F-actin, mounted in 2% rhodamine phalloidin (Molecular Probes) in PME buffer and incubated 50 min in dark before imaging. To assess SAB-3xYpet localization relative to PPB, two sections (one through the middle of the cell and one 4–5 μm apart) were evaluated. Lambda scan of root hair initiation sites Lambda scans of trichoblasts undergoing hair initiation were captured from live Col-0 seedlings and seedlings expressing SAB-3xYpet, using a Zeiss LSM780 confocal microscope. On excitation at 514 nm, 32 images were acquired with narrow detection windows covering the spectral region between 416 nm and 686 nm, in Z stacks of planes at a distance of 2 μm. Maximum intensity Z projections were generated and lambda stacks were visualized in wavelength-coded colour view employing ZEN2010 (Zeiss) software. Statistical analysis Positioning of root hairs, ROP or PIP5K3-YFP patches along trichoblasts, and cell division and microtubule orientation angles did not follow a normal distribution. Thus, significance of differences between distributions was tested with non-parametric, two-sample Kolmogorov–Smirnov test ( http://www.physics.csbsju.edu/stats/KS-test.n.plot_form.html ), which considers both distributions’ location and shape. Distributions of n =150 or 50 trichoblasts from root hair and ROP or PIP5K3-YFP position measurements, respectively, of n =60 cells per mitotic stage, and of n =673–802 or 578–520 cortical microtubules were analysed with significance level P <0.05. Differences in trichome orientation were analysed by F-test (Microsoft Excel), with n =174. Measurements of GFP-BASL polar localization and trichome branching were analysed by Fisher’s exact test ( http://www.quantitativeskills.com/sisa/statistics/fiveby2.htm ), with populations of n >187 and n >400, respectively, with significance level P <0.05. Analysis of trichoblast length was performed by two-tailed, unpaired t -test with equal variance (computed with Microsoft Excel), with n =3 average values of independent experiments and significance level P <0.05. How to cite this article: Pietra, S. et al. Arabidopsis SABRE and CLASP interact to stabilize cell division plane orientation and planar polarity. Nat. Commun. 4:2779 doi: 10.1038/ncomms3779 (2013).